Pattern of extinction of the woolly mammoth in Beringia Extinction of the woolly mammoth in Beringia has long been subject to research and speculation. Here we use a new geo-referenced database of radiocarbon-dated evidence to show that mammoths were abundant in the open-habitat of Marine Isotope Stage 3 ( ∼ 45–30 ka). During the Last Glacial Maximum ( ∼ 25–20 ka), northern populations declined while those in interior Siberia increased. Northern mammoths increased after the glacial maximum, but declined at and after the Younger Dryas ( ∼ 12.9–11.5 ka). Remaining continental mammoths, now concentrated in the north, disappeared in the early Holocene with development of extensive peatlands, wet tundra, birch shrubland and coniferous forest. Long sympatry in Siberia suggests that humans may be best seen as a synergistic cofactor in that extirpation. The extinction of island populations occurred at ∼ 4 ka. Mammoth extinction was not due to a single cause, but followed a long trajectory in concert with changes in climate, habitat and human presence. Woolly mammoth ( Mammuthus primigenius Blum.) were abundant in Beringia during the late Pleistocene before disappearing in the Holocene, and their extinction remains of wide interest and speculation [1] , [2] , [3] , [4] , [5] , [6] , [7] , [8] , [9] , [10] , [11] , [12] , [13] . The Pleistocene environment they occupied is often referred to as 'mammoth steppe', although the nature and chronology of this habitat has been debated [5] , [9] . Extinction has been attributed to one or a combination [1] , [2] , [5] , [8] of factors including over-hunting by humans [1] , [5] , [7] , [13] , ecological displacement during the transition from the Last Glacial Maximum (LGM) to the warm and stable Holocene [1] , [6] , [7] , [8] , [9] , or impact by an extraterrestrial object [14] at the time of the Younger Dryas (YD) climatic oscillation. We reconstruct the detailed pattern of extinction in Beringia, the last redoubt of the mammoths, and examine these various extinction hypotheses by comparing spatially and temporally the changes in mammoth populations relative to environmental changes over the past 45 ka (45,000 cal. years before present) using a georeferenced radiocarbon database of 1,323 woolly mammoth dates, 658 peatland initiation dates, 447 tree and wood macrofossil dates, 576 dates from Paleolithic archaeological sites ( ∼ 45 ka–10 ka), palynological records and genetic data. Patterns of Mammoth Abundance during MIS 3 Of the 1,323 mammoth radiocarbon dates, 377 are infinite in age or classified as potentially >45 ka. Finite-age mammoth remains are abundant from Marine Isotope Stage 3 (MIS 3), and notably common at northern sites, suggesting more favourable conditions for woolly mammoths in northernmost Asia and adjacent North America between ∼ 30 to 45 ka than during the subsequent LGM ( Figs 1 , 2 , 3 ). Mitochondrial DNA for Siberian woolly mammoths suggests that two distinct clades were extant during MIS 3 (ref. 15 ) ( Supplementary Fig. S1 ). Paleolithic human sites in Asian Beringia and particularly its southern periphery are widely present during MIS 3 and demonstrate a long sympatry between humans and woolly mammoths in that region ( Figs 1 and 2 ). 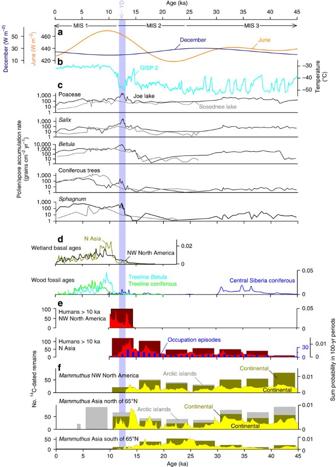Figure 1: Comparative time series of woolly mammoth abundance. Comparative time-series of orbital forcing, environmental factors, Paleolithic human sites and woolly mammoth abundance. (a). General boundaries of marine isotope stages (MIS 1,2,3) and June (orange) and December (dark blue) insolation variations at 60°N. The timing of the YD is indicated. (b). Arctic surface temperatures as represented in Greenland Greenland GISP2 ice core (light blue). (c) Pollen/spore accumulation rates for Poaceae (grass),Salix(willow),Betula(birch), coniferous trees, andSphagnumin northeastern Asia (Sosednee Lake, grey) and Alaska (Joe Lake, black). (d). Radiocarbon age probability plots for wetland/peatland initiation dates (olive green and black), andBetula(birch) (light blue) and treeline conifer macrofossils (lime green). Probability plot of radiocarbon ages from coniferous tree macrofossils from central Siberia is presented in blue. (e) Cumulative probabilities (sum probability in 100-yr periods) of northern Eurasian Paleolithic dates and occupation episodes (blue) per 1,000-year periods and cumulative probabilities of early Alaska-Yukon human occupation sites (red). The cumulative probabilities are overlain on simple histograms of the number of dates per 5,000-year interval (dark red). All human site data series are terminated at 10 ka. (f) Cumulative probabilities of northern Asian and northwestern North American woolly mammoth remains (yellow) overlain on simple histograms of the number of dates per 5,000-year interval (dark yellow). Histograms are divided by continental sites (yellow) and island sites (grey). Histograms are included as cumulative probability curves are prone to age-dependent bias as explained inSupplementary Information. For data sources and calculations, seeMethodsandSupplementary Data 1. Figure 1: Comparative time series of woolly mammoth abundance. Comparative time-series of orbital forcing, environmental factors, Paleolithic human sites and woolly mammoth abundance. ( a ). General boundaries of marine isotope stages (MIS 1,2,3) and June (orange) and December (dark blue) insolation variations at 60°N. The timing of the YD is indicated. ( b ). Arctic surface temperatures as represented in Greenland Greenland GISP2 ice core (light blue). ( c ) Pollen/spore accumulation rates for Poaceae (grass), Salix (willow), Betula (birch), coniferous trees, and Sphagnum in northeastern Asia (Sosednee Lake, grey) and Alaska (Joe Lake, black). ( d ). Radiocarbon age probability plots for wetland/peatland initiation dates (olive green and black), and Betula (birch) (light blue) and treeline conifer macrofossils (lime green). Probability plot of radiocarbon ages from coniferous tree macrofossils from central Siberia is presented in blue. ( e ) Cumulative probabilities (sum probability in 100-yr periods) of northern Eurasian Paleolithic dates and occupation episodes (blue) per 1,000-year periods and cumulative probabilities of early Alaska-Yukon human occupation sites (red). The cumulative probabilities are overlain on simple histograms of the number of dates per 5,000-year interval (dark red). All human site data series are terminated at 10 ka. ( f ) Cumulative probabilities of northern Asian and northwestern North American woolly mammoth remains (yellow) overlain on simple histograms of the number of dates per 5,000-year interval (dark yellow). Histograms are divided by continental sites (yellow) and island sites (grey). Histograms are included as cumulative probability curves are prone to age-dependent bias as explained in Supplementary Information . For data sources and calculations, see Methods and Supplementary Data 1 . 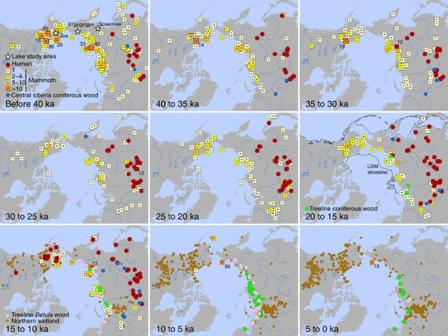Figure 2: Spatiotemporal patterns of woolly mammoth presence. Spatiotemporal patterns of woolly mammoth presence, environmental conditions and Paleolithic human sites. Time-slice maps of radiocarbon-dated mammoth remains (yellow and orange), Paleolithic human sites in northern Eurasia and early human occupation sites in Alaska and Yukon (red), wetland/peatland initiations (tan), andBetula(birch) (pink) and coniferous wood macrofossils from treeline in Eurasia (green) and central Siberia (blue). Stars indicate the location of Lake El'gygytgyn, Sosednee Lake and Joe Lake sites. Total number of dates from sites with >10 mammoth dates for any time-slice are noted. For data sources, seeMethodsandSupplementary Data 1. Full size image Figure 2: Spatiotemporal patterns of woolly mammoth presence. Spatiotemporal patterns of woolly mammoth presence, environmental conditions and Paleolithic human sites. Time-slice maps of radiocarbon-dated mammoth remains (yellow and orange), Paleolithic human sites in northern Eurasia and early human occupation sites in Alaska and Yukon (red), wetland/peatland initiations (tan), and Betula (birch) (pink) and coniferous wood macrofossils from treeline in Eurasia (green) and central Siberia (blue). Stars indicate the location of Lake El'gygytgyn, Sosednee Lake and Joe Lake sites. Total number of dates from sites with >10 mammoth dates for any time-slice are noted. For data sources, see Methods and Supplementary Data 1 . 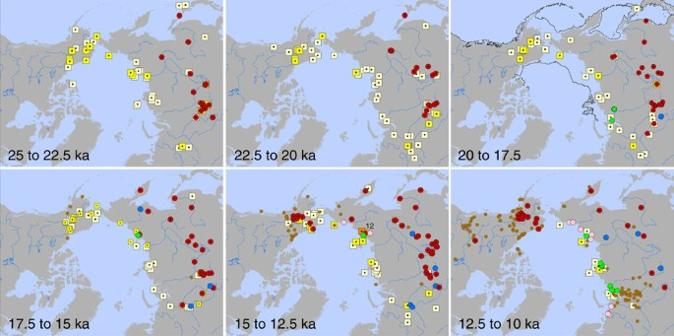Figure 3: Detailed spatiotemporal patterns of mammoth presence and environmental conditions. Detailed spatiotemporal patterns between 25 ka and 10 ka in 2.5 ka time-slices. Time-slice maps and symbols followFig. 2—mammoth,yellow; Paleolithic sites, red; birch macrofossils, pink; interior Siberian conifer wood, blue, treeline conifer wood, green, peatlands/wetlands, tan. Full size image Figure 3: Detailed spatiotemporal patterns of mammoth presence and environmental conditions. Detailed spatiotemporal patterns between 25 ka and 10 ka in 2.5 ka time-slices. Time-slice maps and symbols follow Fig. 2— mammoth,yellow; Paleolithic sites, red; birch macrofossils, pink; interior Siberian conifer wood, blue, treeline conifer wood, green, peatlands/wetlands, tan. Full size image Maximum temperatures in Beringia during MIS 3 were slightly lower (<2 to 3°C) than during the Holocene [16] . June insolation was lower than the Holocene and December insolation was roughly equal ( Fig. 1 ). Northerly areas supported a mosaic of open graminoid and herbaceous vegetation with shrubland. Conifers were present in interior areas [17] , although likely not as abundant as during the Holocene ( Figs 1 and 4 ). A peak in the northern woolly mammoth populations during MIS 3 is consistent with the known ecology of the species and is supported by recent climate suitability modelling [7] . Mammoths were open vegetation-adapted with diets dominated by graminoids and soft-shoots of selected woody plants such as willow ( Salix ) [4] , [9] , [18] . Conifer trees, although found in the stomachs of some woolly mammoths, are not nutritious browse. Birch ( Betula ) can be toxic to cecal digesters, such as mammoths, which lack a rumen for detoxification [5] , [9] , [18] . While grasses and willows were plentiful, birch was less abundant during MIS 3 than its Late Glacial–Holocene maximum [17] ( Figs 1 and 4 ). Northern peatlands would have represented difficult terrain and a poor source of nutrition for mammoths. Relatively low abundances of Sphagnum moss spores in palynological records and a paucity of peat deposits from this period [19] ( Figs 1 , 2 and 4 ) suggest that peatlands were less extensive than during the Holocene. In the north MIS 3, with relatively abundant grass and willow cover, may represent an environment closest to the idealized mammoth steppe. 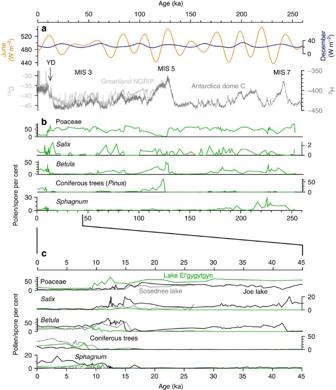Figure 4: Comparative time series of orbital forcing and pollen records from Beringia. Comparative time series of orbital forcing, ice-core climate evidence related to MIS 7–1, and pollen records from Beringia for the past 250 ka and 45 ka. (a) June and December insolation variations at 60°N, general timing of marine isotope stages (MIS 3, 5, 7) and the YD, oxygen-stable isotope record from the Greenland NGRIP ice core, deuterium stable isotope record from the Antarctica Dome C EPICA ice core, (b) Vegetation change in western Beringia over the last∼250 ka as represented by pollen and spore percentages of Poaceae (grass),Salix(willow),Betula(birch), coniferous trees, andSphagnumfrom Lake El'gygytgyn. (c) Vegetation change in eastern and western Beringia for the last 45 ka as represented by pollen and spore percentages of Poaceae,Salix,Betula, coniferous trees, andSphagnumfrom Lake El'gygytgyn and Sosednee Lake, Siberia and Joe Lake, Alaska. For data sources, seeMethods. Figure 4: Comparative time series of orbital forcing and pollen records from Beringia. Comparative time series of orbital forcing, ice-core climate evidence related to MIS 7–1, and pollen records from Beringia for the past 250 ka and 45 ka. ( a ) June and December insolation variations at 60°N, general timing of marine isotope stages (MIS 3, 5, 7) and the YD, oxygen-stable isotope record from the Greenland NGRIP ice core, deuterium stable isotope record from the Antarctica Dome C EPICA ice core, ( b ) Vegetation change in western Beringia over the last ∼ 250 ka as represented by pollen and spore percentages of Poaceae (grass), Salix (willow), Betula (birch), coniferous trees, and Sphagnum from Lake El'gygytgyn. ( c ) Vegetation change in eastern and western Beringia for the last 45 ka as represented by pollen and spore percentages of Poaceae, Salix , Betula , coniferous trees, and Sphagnum from Lake El'gygytgyn and Sosednee Lake, Siberia and Joe Lake, Alaska. For data sources, see Methods . Full size image Declines and shifts in mammoth abundance during the LGM As summer insolation decreased during the LGM (MIS 2), woolly mammoth declined in both northernmost Asia and in northwestern North America ( Figs 1 , 2 , 3 ). The decline in mammoth remains in northern Asia is statistically significant (3-group ANOVA test of mean number of dated samples per 5000 year time period for MIS 3 versus LGM versus Early Postglacial, P <0.05). However, Asian populations overall remained large because of increases in central and southern Siberia. The increase in mammoth remains from the LGM compared with MIS 3 in southerly Siberia is statistically significant (ANOVA P <0.05). Ancient mitochrondial DNA [20] shows that the current genomics data do not offer the resolution required to detect any significant changes in effective population size during the transition from MIS 3 to the LGM ( Supplementary Fig. S1 ). As seen previously [21] , the Bayesian skyline plot (BSP) of available data fails to recover any signature of mammoth decline or eventual extinction. We propose several explanations for this result. First, although the alignment comprises the mitochondrial hypervariable region, which should be the most rapidly evolving region of the mitochondrial genome, very few polymorphisms are observed in the mammoth sample. The data are therefore not sufficiently informative to estimate a mutation rate or to infer the demographic history of the mammoth population without resulting in wide confidence limits. Second, if extinction occurred rapidly, it would be nearly impossible to sample the individuals that would be representative of the few remaining populations. Third, the population structure will also influence the capacity to reconstruct the dynamics of an extinction. If the final few populations of mammoths were geographically isolated and genetically distinct, sampling one or a few individuals from each of these would result in no apparent loss of genetic diversity. In the current analysis, this fragmented landscape scenario may be indistinguishable from a large interbreeding population that remains constant in size. Finally, previous analyses that have used BSPs to infer Pleistocene demographic history used data sampled from populations that experienced a bottleneck and subsequent recovery [22] . Unfortunately, that recovery period may be necessary to capture the dynamics of the population decline. Although the specific timing is uncertain, mitochondrial DNA genologies do show that a northern chromosomal clade of woolly mammoth may have gone extinct during the LGM [15] ( Supplementary Fig. S1 ). Summers in Beringia during the LGM have been estimated to have been 6 °C cooler than present and annual temperatures 4 °C to 12 °C below modern [16] , [23] . Although there was a mosaic of differing land covers, much of the environment was likely cold and dry with large areas of sparse vegetation [5] , [16] , [23] , [24] , [25] . Climatic suitability models predict a sharp decline in woolly mammoth habitat during the LGM [7] . The paleoecological data suggest that rather than a highly productive mammoth steppe of extensive lush grassland supporting large populations of grazers and browsers, at many northern locations, the LGM presented an 'extreme environment' with 'sparse forage' [5] and is associated with mammoth population declines and possibly the loss of one genetic clade [15] in the northern coastal area ( Figs 1 , 2 , 3 , 4 ; Supplementary Fig. S1 ). The increase in mammoth remains and sites from more southerly portions of Siberia, particularly between ∼ 25 and 20 ka, suggest a southward shift in the most favourable mammoth habitat during the LGM. Forest cover declined and this may have provided more open-habitat preferred by mammoths in interior regions ( Figs 1 , 2 , 3 , 4 ). Mammoths also lived south of the the ice sheets in North America during the LGM, but consideration of the taxa there, environmental conditions, the presence or absence of human hunters, and the relative size of mammoth populations is beyond the scope of this paper. Initial resurgence of northern mammoth populations following the LGM As warming progressed following the LGM through the transition from MIS 2 to MIS 1, there was a strong resurgence of woolly mammoth in both northernmost Asia and Alaska/Yukon ( Figs 1 , 2 , 3 ). The increase in mammoth remains in northern Asia and North America following the LGM is statistically significant (ANOVA P <0.05). Across northern Beringia, there were increasing temperatures and a likely increase in the productivity of herbaceous and shrubby vegetation including willows [5] , [25] , [26] , [27] , [28] ( Figs 1 and 4 ). Before the subsequent full development of large peatlands, dense birch cover and conifer forest ( Figs 1 , 2 , 3 , 4 ), these conditions would have promoted woolly mammoth population growth in the north [5] . Populations in southern Siberia were, in contrast, declining relative to LGM levels, probably because of conifer forest and peatland development and possibly greater human hunting pressures ( Figs 1 , 2 , 3 , 4 ). The geographic distribution of the Asian population density was shifting back to a pattern of higher density in the north. However, unlike MIS 3, the more southerly populations seem to have disappeared almost entirely by ∼ 12.5 ka ( Figs 1 , 2 , 3 ). Ultimate decline and Holocene extinction A steep decline in woolly mammoths in northern North America occurred around the time of the YD at ∼ 12.9 ka and in northern Asia, during the subsequent continued development of extensive birch cover, peatlands and conifer forest ( Figs 1 , 2 , 3 , 4 ). Temperature reconstructions suggest a rapid cooling of 3.5 °C to 8.9 °C in portions of Alaska during the YD [29] . However, climatic and vegetation impacts were regionally variable [28] , [29] , [30] , and there is no clear vegetation change in the pollen records, presented here, that can be ascribed to the YD ( Figs 1 and 4 ). Even in the face of vegetation resilience, a very rapid cooling could have been more deleterious to large mammals that remain active year round. Stable isotope studies of woolly mammoth remains suggest that they did not migrate appreciable distances [31] , and confined latitudinal ranges would possibly have made them vulnerable in areas with pronounced cooling. In the absence of information on the specifics of mammoth physiology, the potential impacts of such an oscillation, however, remain uncertain. North American mammoth populations do seem to have declined coincidentally with the YD ( Fig. 1 ), but such a decline is not as clear for Asia. Although it's potential impact on mammoths is still to be resolved, it is notable that a rapid climatic oscillation analogous to the YD does not appear to have occurred during the earlier MIS 6–MIS 5 glacial–interglacial transition [32] through which M. primigenius survived. Dated mammoth remains from after the YD come from northernmost Eurasia and Arctic islands (Continental Northern Asia=5, Arctic Islands=112). Small continental populations of woolly mammoth certainly were present after the YD [6] , [33] , [34] , but trajectory of these populations towards extinction was being driven by changing habitat and perhaps also through human hunting that had spread to North America ( Fig. 3 ). Graminoid, willow and drier herbaceous cover decreased in concert with the establishment of deleterious birch shrubland/woodland throughout Beringia, development of extensive peatlands and wet tundra, and expansion of conifer forest including areas north of the modern treeline across Eurasia as far as the present coastline [5] , [25] , [26] , [27] , [28] , [35] , [36] , [37] ( Figs 1 , 2 , 3 , 4 ). Pressure from hunting was also present, as contemporary Paleolithic sites are numerous in both Siberia and now in northwestern North America ( Figs 1 , 2 , 3 ). Modelling studies show that given the environmental stresses at the time, even limited hunting by humans could have significantly contributed to woolly mammoth extinction [7] . Humans may have been even more widespread by this time than the radiocarbon database of Paleolithic sites captures. Although chronological control of older paleoenvironmental records presents uncertainties, ancestral mammoths had survived decreased grasslands, increased peatlands and extensive birch shrubland and conifer range expansion during the time of MIS 5 (ref. 35 ) ( Fig. 4 ). However, the magnitude of the decrease in grassland and increase of pine during the Holocene and MIS 5 seems to be not typical of the earlier MIS 7 interglacial in northern Asia [35] ( Fig. 4 ). The geographic pattern of Beringian mammoth extinction, seems to be one of the final populations existing on the northern periphery of a once more extensive range [37] ( Figs 2 and 3 ). This pattern is consistent with the open vegetation available on the fringes of the continents and perhaps less intense human hunting there. As sea-level rose during the Late Glacial and Early Holocene, some of these northern mammoth populations were isolated on what became Wrangel Island and the Pribilof Islands [10] , [11] , [12] . The last surviving mammoths on Wrangel Island may have been driven to extinction by stochastic factors related to their being a small and isolated population, hunting by newly arrived humans or disease [38] . They may also have been affected by cooling during the Neoglacial, which is evident in treeline retreat across northern Eurasia at ∼ 4 ka (ref. 36 ). Unfortunately, it seems that no mammoths were left on continental Asia to take advantage of opening of vegetation as treeline retreated after 4 ka. Not one, but several factors would have made the present interglacial particularly challenging for woolly mammoths in Beringia: the preceding declines in northern populations during the LGM; the rapid and relatively early development of unpalatable birch shurbland; wet tundra and extensive peatlands/wetlands followed by the expansion of conifer forest and woodland to the continental margins in Eurasia; the presence of modern humans not only in Siberia, but now also in North America; and the sudden, but regionally differing, impacts of the YD oscillation. The relative importance of these specific forces may never be wholly resolvable, and was likely regionally variable, but combined, they provided the lethal intersection [1] of factors to drive the woolly mammoths to extinction in continental Beringia with relictual populations hanging on for several millennia on isolated Arctic islands. That final extinction of the island populations signalled the conclusion of the long sunset of the woolly mammoths in Beringia after over 20,000 years of multiple environmental challenges related to changes in climate, habitat and human predation. Radiocarbon dating Radiocarbon date sources and details of all dated mammoth samples are provided in Supplementary Data 1 . Radiocarbon dates from remains of M. primigenius ( n =1323), Paleolithic archaeological sites ( n =576), basal ages of wetland peat deposits within 750 km of woolly mammoth remains ( n =658), wood macrofossils from treeline and central regions of Siberia ( n =447) and Beringia lake sediments ( n =19) were calibrated and reported as ka (thousands of years before AD 1950), using the IntCal09 dataset [39] in CALIB. Dates without specific geo-references, laboratory numbers were excluded. We consider radiocarbon dates ≥42,000 14 C yr BP as potentially >45 ka owing to uncertainties in processing, measurement and calibration of old samples [19] , [39] , [40] . We believe that given the size and geographic extent of the mammoth data set that large changes in the number of dated samples reflects general trends in mammoth abundance [2] . We do not, however, affix any interpretation to finer features such as intermillennial variations in sample numbers. Analysis of the calendar age-range of the 2-σ probability distribution of the uncertainty of the age of radiocarbon-dated mammoth remains (measurement and calibration uncertainty) shows increasing magnitude with age. This is particularly acute for time periods earlier than 15 ka ( Supplementary Fig. S1 ). Simple sums of the number of age-probability distributions that intersect a given time period are thus age-biased and would over estimate abundances for time periods beyond 15 ka. Therefore, mammoth dates are presented as both simple histograms of the number of mammoth dates (medians of calibrated probability distributions) per 5,000-year interval and the cumulative sum of the total calibrated probability distributions (cumulative probability) in 100-yr periods. Care must be taken in the use of large radiocarbon data sets, and debate exists over the best approaches [41] , [42] , [43] , [44] . We have avoided known apatite bone dates for mammoths ( Supplementary Data 1 ), attempted to select archaeological dates with clear context and further mitigate problems in the dating of Asian sites by using occupation-age estimates (see below) that are often based on multiple dates, and we have only incorporated dates from laboratories that we believe participated in either international or internal Soviet/Russian multi-lab intercomparisons. Although issues may still persist with individual dates, we believe the total numbers, incorporated in the analysis, portray overall general records of abundance and geographic patterns with acceptable fidelity. Archaeological dates and Eurasian occupation episodes The dates for Paleolithic sites are from a number of sources [5] , [45] , [46] , [47] , and those from Eurasian Paleolithic sites were used to calculate occupation-episode estimates for 1,000-year time-slices to remove any bias introduced by sites that have many dates for a single occupation period owing to the employed sampling and dating methods [45] , [46] , [47] . The occupation episode totals for each time-slice represent the number of geographically discrete sites that have dates indicating human presence during that time period. Other paleoenvironmental data sets and chronologies Online data for June and December insolation variations at 60°N (ref. 48 ), temperature and oxygen stable isotope records from the Greenland GISP2 and NGRIP ice cores [49] , [50] , deuterium stable isotope record from the Antarctica EPICA Dome C ice core [51] and the pollen and spore data for the Joe Lake and Sosednee Lakes cores [52] , [53] were obtained from the NOAA National Climate Data Center site ( www.ncdc.noaa.gov/paleo ). Additional data for Sosednee Lake were provided by Dr Pat Anderson. Chronologies were constructed by fitting a cubic spline to the sediment age-depth relationship based on calibrated [39] radiocarbon dates. Pollen and spore concentrations for Lake El'gygytgyn were received in digital format courtesy of Drs Anatoly Lozhkin and Pat Andersen and are from 2005. As presented, they may differ slightly in terms of pollen sum used to calculate percentages, details of counts and subsamples represented in previously published form [35] . There has been previous discussion regarding the chronology for Lake El'gygytgyn [35] , [54] , [55] , and we use an updated chronology incorporating orbital tuning provided by Drs Norbert Nowaczyk and Julie Brigham-Grette. Peat/wetland initiation and wood macrofossil dates are from several sources [19] , [36] , [56] , [57] . Bayesian skyline plots BSPs ( Supplementary Fig. S1 ) were reconstructed for a data set of 103 mammoth mitochondrial control region sequences, comprising all currently available sequence data [20] , [58] . Analyses were performed in BEASTS [59] , [60] using the HKY+G model of nucleotide substitution and calibrated radiocarbon dates to constrain the molecular clock. The significance of the downward trend in diversity was investigated using Bayes Factors [60] to compare two different coalescent priors: the flexible BSP [58] and a constant-size coalescent prior. The BSP is a piecewise-constant coalescent model, in that it allows several different constant population sizes to have existed throughout the sampled evolutionary history (in this case ten different population sizes), and then averages these estimates across the a posteriori sampled trees. For each analysis, two Monte Carlo Markov chains were run for 30 M iterations, with samples drawn from the posterior every 3,000 iterations. After checking for appropriate mixing and convergence, the first 10% of samples from the posterior were discarded and the remainder combined. BSPs and Bayes Factorss were estimated using Tracer v 1.5 [61] . How to cite this article: MacDonald, G.M. et al . Pattern of extinction of the woolly mammoth in Beringia. Nat. Commun. 3:893 doi: 10.1038/ncomms1881 (2012).